Self-assembled tunable networks of sticky colloidal particles Surfaces decorated with dense arrays of microscopic fibres exhibit unique materials properties, including superhydrophobicity and low friction. Nature relies on ‘hairy’ surfaces to protect blood capillaries from wear and infection (endothelial glycocalyx). Here we report on the discovery of self-assembled tunable networks of microscopic polymer fibres ranging from wavy colloidal ‘fur’ to highly interconnected networks. The networks emerge via dynamic self-assembly in an alternating electric field from a non-aqueous suspension of ‘sticky’ polymeric colloidal particles with a controlled degree of polymerization. The resulting architectures are tuned by the frequency and amplitude of the electric field and surface properties of the particles. We demonstrate, using atomic layer deposition, that the networks can serve as a template for a transparent conductor. These self-assembled tunable materials are promising candidates for large surface area electrodes in batteries and organic photovoltaic cells, as well as for microfluidic sensors and filters. Surfaces patterned with micro-scale fibres are attracting enormous attention for their unique features [1] , [2] , [3] , [4] , [5] , including self-cleaning [6] , anti-biofouling [7] and superhydrophobicity [8] . Materials based on the arrays of flexible synthetic pillars immersed in soft gels exhibit homeostatic self-regulating properties and adaptivity [1] . Most of these patterned surfaces are engineered by top-down methods, e.g., soft lithography [9] . A large number of diverse patterning techniques, which use organic and polymeric materials, including solvent-assisted micro-molding [10] , micro-contact printing [11] and dip-pen nanolithography [12] , form the basis of contemporary soft lithography. Design of the nontrivial three dimensional (3D) structures via bottom-up methods such as self-assembly [13] , [14] , [15] and surface instabilities [16] are highly desirable but technically challenging. For instance, electrohydrodynamic instability [17] may yield 3D patterns at the interface between liquid dielectric materials without a pre-patterned mask. However, the progress is impeded by low controllability and irreproducibility of the emerging structures. External electric/magnetic fields are often used to promote colloidal self-assembly [18] , [19] or form colloidal chains in electro- and magneto-rheological fluids along the direction of an applied field [20] , [21] . Nontrivial structures can be generated in suspensions of metallo-dielectric patchy and dumbbell particles in external alternating electric or magnetic fields [22] , [23] , [24] , [25] . However, these structures tend to disassemble as soon as the field is turned off unless fixed by crosslinkers [26] . Recently developed methods of thermal annealing of colloidal patterns allow fixing some of the field-generated assemblies of spherical particles [27] , [28] . Another promising alternative to the lithographic methods is a dynamic self-assembly [29] occurring in out-of-equilibrium conditions. For example, dynamic self-assembly allows the formation of diverse functional structures from suspensions of colloidal particles. The structures, which generally do not exist under equilibrium conditions, include radial magnetic asters [30] , dynamic swimmers [31] , self-healing membranes [32] , particle foams [33] , self-assembled microtubes [34] and binary linear clusters [35] . Here we report on self-assembly of sticky colloidal particles energized by an ac electric field. The system generates permanent and tunable structures that can be used as templates for 3D fabrication. Our system is comprised of a colloidal suspension of epoxy polymer/hardener mixture in a dielectric organic solvent (toluene) confined in a thin electric cell. The suspension is energized by a uniaxial alternating electric field (see Methods). The field also provides a convenient mean to control the emergent architectures. The resulting behaviour is further tuned by varying the polymerization time of epoxy polymer/hardener mixture before the solvent, quenching the polymerization, is introduced. Select results featuring dense wavy arrays of self-assembled colloidal fibres (colloidal fur) and permanent interconnected networks are displayed in Fig. 1 . These structures can further be used as motifs for specific functionalization or coating, e.g., by atomic layer deposition (ALD). 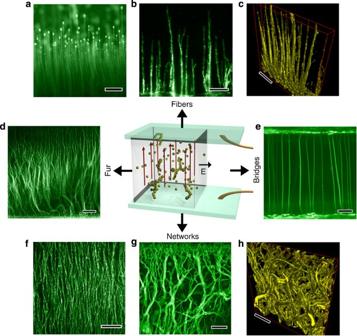Figure 1: Self-assembled structures formed by sticky epoxy particles. Image in the center illustrates the schematics of the experiment. (a) Reversible self-assembled polymer fibres (‘mushrooms’) formed at a low degree of polymerization. Array of fibres grows from the electrode surface along the appliedacelectric field (50 Hz, 700 V) and form pillars with a pearl at the end. Scale bar is 20 μm. (b) Permanent self-assembled polymer brushes (‘hair’) formed by the sticky particles with a high degree of polymerization in the electric field of 100 Hz, 1 kV. Fibres comprised of individual particles that form permanently bonded chains along the electric field direction. Scale bar is 20 μm. (c) 3D reconstruction of a permanent self-assembled array of polymer fibres from the stacks of 2D confocal images. Fibres densely cover the surface of the electrode. Scale bar is 20 μm. (d) Colloidal fur is formed from highly polymerized colloidal epoxy particles in low frequency applied electric field (50 Hz, 800 V shown). Scale bar is 100 μm. (e) Retractable polymer fibres form multiple bridges connecting opposite electrodes withacelectric field values of 1 Hz, 1 kV. Scale bar is 100 μm. (f) A network of interconnected chains of sticky colloidal particles with a high degree of polymerization is formed for 900 Hz and 700 V. Scale bar is 30 μm. (g) A network of bundled chains of sticky particles (gel) is formed at 200 Hz 700 V. Scale bar is 50 μm (h) 3D reconstruction of the network of interconnected polymer chains from the stacks of 2D confocal images for the same parameters as in (g). Scale bar is 20 μm. Figure 1: Self-assembled structures formed by sticky epoxy particles. Image in the center illustrates the schematics of the experiment. ( a ) Reversible self-assembled polymer fibres (‘mushrooms’) formed at a low degree of polymerization. Array of fibres grows from the electrode surface along the applied ac electric field (50 Hz, 700 V) and form pillars with a pearl at the end. Scale bar is 20 μm. ( b ) Permanent self-assembled polymer brushes (‘hair’) formed by the sticky particles with a high degree of polymerization in the electric field of 100 Hz, 1 kV. Fibres comprised of individual particles that form permanently bonded chains along the electric field direction. Scale bar is 20 μm. ( c ) 3D reconstruction of a permanent self-assembled array of polymer fibres from the stacks of 2D confocal images. Fibres densely cover the surface of the electrode. Scale bar is 20 μm. ( d ) Colloidal fur is formed from highly polymerized colloidal epoxy particles in low frequency applied electric field (50 Hz, 800 V shown). Scale bar is 100 μm. ( e ) Retractable polymer fibres form multiple bridges connecting opposite electrodes with ac electric field values of 1 Hz, 1 kV. Scale bar is 100 μm. ( f ) A network of interconnected chains of sticky colloidal particles with a high degree of polymerization is formed for 900 Hz and 700 V. Scale bar is 30 μm. ( g ) A network of bundled chains of sticky particles (gel) is formed at 200 Hz 700 V. Scale bar is 50 μm ( h ) 3D reconstruction of the network of interconnected polymer chains from the stacks of 2D confocal images for the same parameters as in ( g ). Scale bar is 20 μm. Full size image Self-assembly at low degree of polymerization At a low degree of polymerization the epoxy polymer/hardener mixture (below 3 min., see Methods) gives rise to liquid-like colloidal particles that produce smooth fibre structures when subjected to the ac electric field. Parallel retractable polymer fibres are formed at the electrode surfaces along the applied electric field. Depending on the parameters of the electric field, dynamic brushes of fine soft fibres, as seen in Fig. 1a , or bridges spanning the electrodes ( Fig. 1e ) are formed. Higher frequencies promote short, fine fibres while low frequencies result in long fibres gradually coalescing to thicker structures ( Fig. 1e ). Increasing the amplitude of the applied field favours more extended fibres. Self-assembly at high degree of polymerization At a higher degree of polymerization the mixture gives rise to ‘sticky’ colloidal particles formed by epoxy polymers that are partially cross-linked to a higher degree than in a liquid-like colloid (see Methods). These sticky particles self-assemble into permanent structures. A few examples are shown in Fig. 1b,d,f,g . Triggered and controlled by the external ac electric field at elevated frequencies (about 100 Hz), the system self-assembles to colloidal ‘fur’: a dense brush of wavy fibres, see Fig. 1d . In this case, the field-induced hydrodynamic flow of the solvent is low and local arrangement of the polarizable particles is governed mostly by the head-to-tail electrostatic interactions. As we decrease the frequency, the hydrodynamics of the solvent comes into play, promoting the formation of wavy fibres. Furthermore, depending on the parameters of the ac field, sticky epoxy particles assemble into interconnected chains ( Fig. 1f ) or tightly bundled networks of glued particles ( Fig. 1g ). Tunable liquid-like fibres comprised of particles with a low degree of polymerization reversibly extend and retract in response to the ac electric field. The growth of these fibres proceeds via successive coalescence of the colloidal droplets connected to the electrode. The droplets, moving in response to the electric field, form mushroom-like pillars with a distinctive pearl at the tips (as shown in Figs 1a and 2c ). 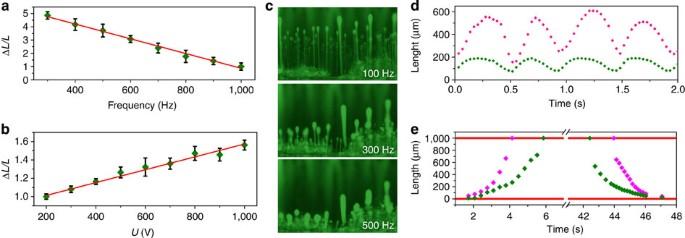Figure 2: Retractable fibres forming from liquid-like particles with low degree of polymerization. (a) Frequency dependence of the fibres’ relative length (ΔL/L) (1 kV). (b) Relative length (ΔL/L) as a function of the applied voltage, frequency 100 Hz. The error bars are standard deviations of the measured values. (c) Optical fluorescent images of the fibres at different frequencies. (d) Fibre length as a function of time at 1 Hz and 1 kV for short and long ‘mushroom’ fibres. For both fibres, an almost complete reversibility is observed after multiple extension/retraction cycles during 30 min. (e) Time dependence of the fibre length during the formation of the bridges between opposite electrodes, frequency 0.1 Hz. Figure 2a,b illustrates the frequency and voltage dependence of the fibres’ relative length (Δ L/L ). The trend for both dependences is close to linear: the fibres’ length increases with the increase of the applied voltage and with the decrease of the frequency. Optical fluorescence images of the fibres at different frequencies are shown in Fig. 2c . Being fully reversible, the pillars periodically extend and retract at low frequency (1 Hz) of the ac field, see Fig. 2d . Bridges (1,000 μm long fibres) traversing the electrodes of the cell are formed upon application of longer voltage pulses, Fig. 1e . The rate of bridge formation depends on the amount of locally available colloidal material, Fig. 2e . Figure 2: Retractable fibres forming from liquid-like particles with low degree of polymerization. ( a ) Frequency dependence of the fibres’ relative length (ΔL/ L ) (1 kV). ( b ) Relative length (ΔL/ L ) as a function of the applied voltage, frequency 100 Hz. The error bars are standard deviations of the measured values. ( c ) Optical fluorescent images of the fibres at different frequencies. ( d ) Fibre length as a function of time at 1 Hz and 1 kV for short and long ‘mushroom’ fibres. For both fibres, an almost complete reversibility is observed after multiple extension/retraction cycles during 30 min. ( e ) Time dependence of the fibre length during the formation of the bridges between opposite electrodes, frequency 0.1 Hz. Full size image Sticky colloidal particles, comprised of epoxy droplets of a higher degree of polymerization, exhibit a surprisingly rich morphology of permanent fibrilous structures formed in an ac electric field. With the increase in the frequency of the ac field, bundled wavy fibres, formed in the conditions where hydrodynamic flows are important, give way to highly interconnected single-particle thick networks ( Fig. 3c ), and then to parallel chains of permanently bonded particles ( Fig. 3d ). Hydrodynamic flow of the solvent is negligible in the later cases. The dynamics of the bundled phase is rather nontrivial. Upon application of the ac electric field, particles self-assemble into parallel chains oriented along the field direction. Then the onset of the hydrodynamic flow takes place and the system forms bundles of wavy chains (see Supplementary Movie 1 ). 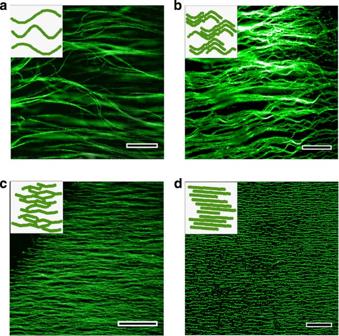Figure 3: Self-assembled structures formed from highly polymerized sticky particles. (a) Colloidal fur formed by permanently bonded particles that self-assembled into long wavy chains at low frequencies of the applied field. For these parameters of theacelectric field, hydrodynamic flow is responsible for the formation of wavy structures (50 Hz, 1 kV shown). Scale bar is 100 μm. (b) Wavy bundled chains (chevrons) of sticky colloidal particles are formed in a large range of frequencies and voltages and are also affected by the hydrodynamic flow around the chains (300 Hz, 1 kV is displayed). Scale bar is 100 μm. (c) Interconnected permanently bonded chains assembled along the electric field at 700 Hz, 1 kV. (d) Individual chains of colloidal particles along 1,000 Hz, 1 kV electric field. Scale bar is 50 μm. Figure 3: Self-assembled structures formed from highly polymerized sticky particles. ( a ) Colloidal fur formed by permanently bonded particles that self-assembled into long wavy chains at low frequencies of the applied field. For these parameters of the ac electric field, hydrodynamic flow is responsible for the formation of wavy structures (50 Hz, 1 kV shown). Scale bar is 100 μm. ( b ) Wavy bundled chains (chevrons) of sticky colloidal particles are formed in a large range of frequencies and voltages and are also affected by the hydrodynamic flow around the chains (300 Hz, 1 kV is displayed). Scale bar is 100 μm. ( c ) Interconnected permanently bonded chains assembled along the electric field at 700 Hz, 1 kV. ( d ) Individual chains of colloidal particles along 1,000 Hz, 1 kV electric field. Scale bar is 50 μm. 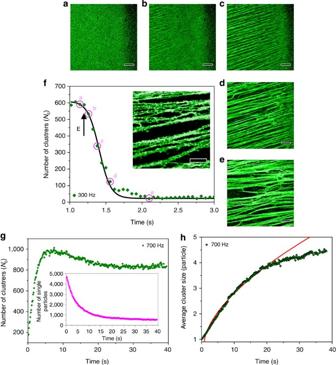Figure 4: Bundled individual and interconnected chains of sticky particles at 300 and 700 Hz. (a–e), Sequence of snapshots illustrating self-assembly of bundled chains from a suspension of sticky particles. Approximately 0.5 s after application of the field (300 Hz, 1 kV), individual particles are absorbed by short chain segments. Scale bar is 50 μm. (b,c) Self-assembly proceeds via propagation of the front. Hydrodynamic flow triggers deformation of the bundled chains, which finally form a permanent structure. (f) Time dependence of the number of clusters. Initial slow growth of short chains is followed by a fast interconnection event (gelation). The line is a guide for the eye. The arrow indicates the moment when the electric field is turned on. The inset shows the network of close-packed chains. Scale bar is 20 μm. (g) Time dependence of the total number of clusters,Nc, for 700 Hz and 1 kV. Initial linear increase, corresponding to the formation of individual chains, is followed by the decrease due to fusions and interconnections between the chains. The inset illustrates the decay of the number of single particles. (h) Time evolution of the average cluster size. The solid line is a power-law fit ~t0.6. Full size image Figure 4a–e illustrates consecutive formation of bundled chains starting from a single-particle sticky colloidal suspension. Time evolution of the number of clusters (chain segments) for the frequency of 300 Hz is shown in Fig. 4f . Initially slow growth of short chains is replaced by a fast interconnection event (gelation transition, around 1 s in the graph). Gelation results in a formation of giant clusters comprised of long bundled chains spanning both electrodes. The dynamics can be further tuned by the frequency. Time evolution of the number of clusters N c (chain segments containing at least two colloidal particles) at 700 Hz is shown in Fig. 4g . For this frequency a complete gelation does not occur. The initial increase of N c corresponds to the formation of permanent individual chains that are aligned along the field direction. The initial trend is close to a linear law. That differs from the known exponent for the average chain length ζ =0.6 (ref. 36 ) because the monomers (single particles) are excluded from the analysis. According to the Smoluchowski coagulation theory [37] , the initial growth of the multi-particle clusters from a single-particle state is linear. Then, the curve exhibits a decrease in N c corresponding to the onset of fusion and interconnections between the chains. The inset to Fig. 4g confirms that the number of single particles decay with time. Evolution of average cluster size versus time is shown in Fig. 4h . In this case, the behaviour is consistent with a power law with the exponent ζ =0.6 (ref. 26 ), although the scaling interval is relatively short due to limited statistics. Similar behaviour is observed for higher frequencies. However, the overall self-assembly time-scale increases with the increase in frequency, likely due to the decrease of the double layer polarization [38] . The frequency f 0 of the gelation transition can be estimated from the characteristic time t 0 for the ions in solvent to diffuse a distance of the order of the Debye length λ D ~2–2.5 μm, i.e., f 0 =1/ t 0 = D / λ D 2 ~250–300 Hz (where D ~10 −9 m 2 s −1 is the ion’s diffusion, see Methods). Above this value polarization of the double layer becomes small, resulting in attenuation of the inter-particle dipolar interaction. Furthermore, the flows induced by particles’ oscillations in the ac field that are responsible for the formation of fur and bundled chains subside with the increase of the frequency. Using measured values of the electrophoretic mobility μ e ~3-4 × 10 −10 m 2 V s −1 and applied electric field E =10 6 V m −1 (see Methods), we can estimate the frequency, f c , when the induced flows become negligible, i.e., when the displacement is comparable to the particle radius R , yielding f c = μ e E /( 2 π R) ~50–60 Hz. This range is in good agreement with the onset of fur formation at 50 Hz. Figure 4: Bundled individual and interconnected chains of sticky particles at 300 and 700 Hz. ( a – e ), Sequence of snapshots illustrating self-assembly of bundled chains from a suspension of sticky particles. Approximately 0.5 s after application of the field (300 Hz, 1 kV), individual particles are absorbed by short chain segments. Scale bar is 50 μm. ( b , c ) Self-assembly proceeds via propagation of the front. Hydrodynamic flow triggers deformation of the bundled chains, which finally form a permanent structure. ( f ) Time dependence of the number of clusters. Initial slow growth of short chains is followed by a fast interconnection event (gelation). The line is a guide for the eye. The arrow indicates the moment when the electric field is turned on. The inset shows the network of close-packed chains. Scale bar is 20 μm. ( g ) Time dependence of the total number of clusters, N c , for 700 Hz and 1 kV. Initial linear increase, corresponding to the formation of individual chains, is followed by the decrease due to fusions and interconnections between the chains. The inset illustrates the decay of the number of single particles. ( h ) Time evolution of the average cluster size. The solid line is a power-law fit ~ t 0.6 . Full size image Upon removal of the ac electric field, the particles remain in mechanical contact to each other and the total structure stays intact. The mechanical contacts between the individual particles in the chain were confirmed by scanning electron microscopy (SEM) studies (see Methods). 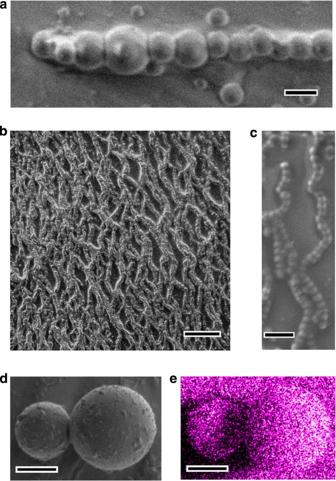Figure 5: SEM study of polymer colloidal chains coated by SnO2using atomic layer deposition. (a) SEM image of the polymer wavy chain formed by spherical colloidal particles. Scale bar is 2 μm. (b) SEM image of the network of interconnected polymer chains. Scale bar is 50 μm. (c) SEM image of the polymer chain formed by permanently bonded colloidal spheres ALD coated with SnO2. Scale bar is 10 μm. (d,e) SEM and EDX (Sn L-edge) mapping of individual colloidal particles uniformly coated with SnO2. Scale bar is 1 μm. Figure 5a,b shows SEM images of a self-assembled chain and a network comprised of the spherical epoxy particles bonded together. Clearly, epoxy colloidal particles have a tendency to partially interpenetrate each other during the assembly process, creating tight mechanically stable bonding that survives capillary forces during solvent evaporation. Figure 5: SEM study of polymer colloidal chains coated by SnO 2 using atomic layer deposition. ( a ) SEM image of the polymer wavy chain formed by spherical colloidal particles. Scale bar is 2 μm. ( b ) SEM image of the network of interconnected polymer chains. Scale bar is 50 μm. ( c ) SEM image of the polymer chain formed by permanently bonded colloidal spheres ALD coated with SnO 2 . Scale bar is 10 μm. ( d , e ) SEM and EDX (Sn L-edge) mapping of individual colloidal particles uniformly coated with SnO 2 . Scale bar is 1 μm. Full size image In order to functionalize the self-assembled structures, we employed ALD to coat the polymer surface of the networks with a thin layer (12 nm) of tin oxide (SnO 2 ). This coating was chosen for its ease of deposition and potential applications in optoelectronics and sensors [39] . SEM images of polymer chains in the network and individual particles that are coated with SnO 2 are shown in Fig. 5 . Thermal stability of the epoxy allowed preservation of the self-assembled structures during the deposition cycles in the ALD chamber at 100 °C. We performed an energy-dispersive X-ray (EDX) mapping of Sn (see Methods) on individual colloidal particles, Fig. 5e . The mapping confirmed uniform coating of the networks with SnO 2 . It provided a proof of concept that the self-assembled networks of sticky polymer colloidal particles can be used as a low-cost alternative for 3D templating. In conclusion, we have demonstrated that sticky polymer colloids in non-aqueous solution form a variety of self-assembled structures, ranging from tunable fibres and bridges to permanent colloidal fur and networks of interconnected, bundled chains. The morphology of these self-assembled structures is controlled by the parameters of the applied electric field and the degree of epoxy polymerization. Our work provides an insight into the engineering of permanent and tunable complex networks by the means of out-of-equilibrium self-assembly. Moreover, this approach is a low-cost alternative to more traditional lithographic techniques. Self-assembled networks of sticky polymer colloids can be further functionalized by the means of ALD and can be used in a wide range of applications where a large surface to volume ratio is needed, such as electrodes in lithium batteries, photovoltaic cells, sensors and filters. Colloidal particle synthesis The precursor was prepared by macroscopic mixing for 1 min of 100 mg of epoxy polymer (bisphenol A diglycidyl ether) and 100 mg of hardener (2,4,6-tris[(dimethylamino)methyl]phenol). Colloidal solutions were made by quenching the polymerization with toluene (anhydrous, water <0.2%) as the solvent and with rhodamine-B-isothiocyanate (RBI) as a tracer dye. Two hundred microlitres of toluene/RBI (1 mg of RBI) solution was introduced in 40 mg of polymer/hardener mixture at a specific time, which is defined as the ‘polymerization’ time, usually in the range from 1 to 5 min measured from the precursor formation. Humidity of the environment was around 60%. Both epoxy polymer and hardener are soluble in toluene, although the hardener has a higher solubility in toluene than the epoxy polymer [40] , [41] , [42] . The mechanism of colloid formation from the epoxy/hardener mixture in toluene is as follows: upon mixing both components (epoxy polymer and the hardener), crosslinking is initialized in multiple random locations of the mixture, giving rise to multiple nuclei of a cross-linked phase. The mixture turns solid after 10 min. The fully cross-linked phase is insoluble in toluene. Placing the polymer/hardener mixture into toluene solvent before a complete cure quenches further crosslinking, and remaining free epoxy and hardener molecules are transferred to the solvent. Consequently, a suspension of microscopic particles comprised of insoluble partially cross-linked epoxy molecules is formed. Average particle size is determined by the time the mixture was exposed to crosslinking before the introduction of the solvent (toluene). Fourier transform infrared spectroscopy characterization Fourier transform infrared spectroscopy (FTIR) was used to characterize the degree of polymerization of epoxy colloidal solutions at different polymerization times. The degree of crosslinking between epoxy polymer and hardener was investigated in the middle range of IR light (Nicolet FTIR spectrometer 6,700). The measurements were carried out on three epoxy colloidal samples (using liquid transmission cells with KBr windows) prepared at 1, 3 and 5 min of polymerization time. Each sample was used after waiting 10 min to allow the sedimentation of oversized colloidal particles. Two well-resolved characteristic absorption bands of the oxirane group, which are impacted by the crosslinking process, are observed in the middle IR (see Supplementary Fig. 1 ). The first band, centred at 918 cm −1 , is attributed to the C-O-C asymmetric stretching of the oxirane group. The second band is centred at ~1,250 cm −1 and is attributed to the C-O-C symmetric stretching of the oxirane group [43] , [44] . The FTIR spectra were normalized to 1,608 cm −1 which is the band corresponding to C=C stretching of the aromatic rings. The changes in these two bands at 918 cm −1 and 1250, cm −1 reveal the opening of the epoxy oxirane rings during crosslinking. The IR spectra also display a pronounced broad band around 3,400 cm −1 , indicative of the formation of the OH groups when crosslinking has occurred [45] . The FTIR analysis confirms that toluene quenches the crosslinking processes. Consequently, particles with a different degree of polymerization are formed depending on the time when the toluene was introduced (see Supplementary Fig. 1 for the FTIR spectra). It is worth noting that the FTIR bands corresponding to H 2 O molecules are not observed, which indicates the absence of moisture absorption by the colloidal samples. In order to gain an insight into ‘sticky’ properties of epoxy colloidal particles, the initial reaction solution was washed to extract epoxy colloidal particles and discard free epoxy and hardener molecules. The colloidal solution was prepared with 200 μl of Toluene/RBI solution mixed with 40 mg of blended epoxy/hardener mixture for different times of polymerization (3 and 5 min). After waiting 10 min for sedimentation (to separate oversized particles), 150 μl of the colloidal suspension was extracted and redispersed in 200 μl toluene, gently centrifuged (500 r.p.m., 10 min) and 200 μl of the media was discarded. This procedure was repeated three times to guarantee an effective purification. The FTIR analysis confirmed that epoxy colloidal particles themselves contain both cross-linked epoxy and active uncross-linked epoxy groups (see Supplementary Fig. 2 ). We separated oversized colloidal particles by 10 min of sedimentation in toluene before the use of the resulting suspension in the electric cell. Particles with low polymerization time (1 min) had an average size of 1.12 μm with size polydispersity of 32% (from light scattering and optical microscopy measurements), whereas particles at high polymerization time (5 min) had a size of 1.94 μm and size polydispersity of 15% (see Supplementary Fig. 3 ). Electric cell The electric cell was comprised of two 100 μm thick copper electrodes glued to a microscope glass slide at a distance of 1 mm and covered with a 0.1 mm thick glass cover slip to form a channel. After a colloidal suspension was introduced into the cell, it was sealed on both sides by Super Silicone Sealant, 3 M. The amplitudes of a single axis ac electric field applied to the cell were in the range from 0 to 1,000 V and the frequencies from 1 mHz to 1 MHz. Electrophoretic mobility and electrical conductivity We determined the particle charge at different degrees of polymerization by means of electrophoretic measurement (zeta-potential analyzer Malvers Nano-ZS) in toluene/RBI mixture. We identified the charge ( Z ) per particle from the electrophoretic mobility ( μ e ) using the relation Z e=6π Rη μ e where R is the particle radius, η is the solvent viscosity ( η =5.9 × 10 −4 Pa s) and e is the electron charge. Average charge per particle Z in electrons varies from 3.3 for 1 min polymerization time to 28.3 for 5 min (see Supplementary Fig. 4 ). For fixed polymerization time, the charge on a colloidal particle is proportional to its surface area ( Supplementary Fig. 5 ). We estimated the Debye screening length ( λ D ) from measurements of the solvent conductivity ( σ ) (toluene/RBI mixture) in the presence of colloidal particles; a single ionic charge was assumed for simplicity. The Debye length was determined as λ D =(ε 0 ε r D / σ) 1/2 , where D is the ion diffusion coefficient ( D =10 −9 m 2 s −1 is a representative value for ion diffusion) and σ is the conductivity of the solvent. The Debye screening length was estimated to be of the order 2 μm with a slight change from 2.15 to 2.57 μm with the increase of the polymerization time from 1 to 5 min (see Supplementary Fig. 6 ). Visco-elasticity properties We analysed visco-elasticity properties of the epoxy polymer by the means of rheological measurements using an Anton Paar Physica MCR 301 rheometer. We used oscillatory and rotational mode with a frequency of 10 Hz and strain amplitude of 5% at 25 °C and measured the loss and storage moduli as a function of the polymerization time in the macroscopic epoxy/hardener mixture (no solvent) at different polymerization times (see Supplementary Fig. 7 ). A mixture with a low degree of polymerization (1 min) has a viscosity of 33.3 Pa s and an elasticity of 1.6 Pa s. A higher polymerization (5 min) mixture was observed to have a viscosity and elasticity of 5.7 and 2.7 kPa s, respectively. The ratio between storage (elastic) and loss (viscous) moduli, tan( Φ ), as a function of polymerization time revealed a transition from liquid-like (low tan( Φ ) values) to solid-like behaviour (high tan( Φ ) values) in around 2.5 min (see Supplementary Fig. 7 ). Optical and electron microscopy Confocal microscopy was performed with an Olympus DSU spinning disc confocal module mounted on an Olympus BX61 microscope, equipped with a Hamamatsu EM-CCD C9100 digital camera and LMplanFluorN x10 and LMplanFluorN oil immersed × 60 objectives (Olympus). We used fluorescence excitations for RBI-labeled colloids with a wavelength of 568 nm. 2D images were captured at 1,024 × 1,024 resolution. For the 3D data reconstruction, we recorded stacks of 2D images spaced at 0.5 μm apart. Image and data analysis was performed by ImageJ software and custom scripts. SEM imaging was performed on a JEOL 7500 setup equipped with an EDX detector for chemical analysis. The EDX measurements were carried out in the mapping mode for Sn L-edge signal on the networks of polymer colloidal chains coated with SnO 2 by ALD. Atomic layer deposition SnO 2 film was synthesized by ALD following a previous recipe [46] in the growth chamber of a commercial ALD system (SavannahS100 from Cambridgenanotech). The growth was performed in the self-limiting regime at 100 °C by pulsing sequentially Tetrakis (dimethylamino)Tin (TDMASn) as the Sn source and hydrogen peroxide (H 2 O 2 ) (35% in water) as the oxygen source. The TDMASn precursor was held at 40 °C in a stainless steel Swagelok cylinder during the deposition. The pulse and purge sequence for the TDMASn and H 2 O 2 was as follows: 0.4–60 s and 0.1–60 s, respectively, constitute one deposition cycle. After 125 deposition cycles, the substrates were removed from the ALD chamber and the film thickness was measured with an ellipsometer (model α-SE from Woollam) on witness silicon pieces placed around the microscope glass. The film thickness (12 nm) was uniform within 1% and had a growth rate of 1.0 Å per cycle. We selected this chemistry based on its large ALD window and low temperature range: from 50 to 300 °C, which is compatible with the stability temperature range of most polymers. How to cite this article: Demortière, A. et al. Self-assembled tunable networks of sticky colloidal particles. Nat. Commun. 5:3117 doi: 10.1038/ncomms4117 (2014).